River-margin habitat ofArdipithecus ramidusat Aramis, Ethiopia 4.4 million years ago The nature and type of landscape that hominins (early humans) frequented has been of considerable interest. The recent works on Ardipithecus ramidus , a 4.4 million years old hominin found at Middle Awash, Ethiopia, provided critical information about the early part of human evolution. However, habitat characterization of this basal hominin has been highly contested. Here we present new sedimentological and stable isotopic (carbon and oxygen) data from Aramis, where the in situ , partial skeleton of Ar. ramidus (nicknamed 'Ardi') was excavated. These data are interpreted to indicate the presence of major rivers and associated mixed vegetations (grasses and trees) in adjacent floodplains. Our finding suggests that, in contrast to a woodland habitat far from a river, Ar. ramidus lived in a river-margin forest in an otherwise savanna (wooded grassland) landscape at Aramis, Ethiopia. Correct interpretation of habitat of Ar. ramidus is crucial for proper assessment of causes and mechanisms of early hominin evolution, including the development of bipedalism. Recent work [1] , [2] , [3] on Ardipithecus ramidus in the Middle Awash, Ethiopia ( Fig. 1 ) is a major milestone in palaeoanthropology, particularly for the discovery of the oldest hominin skeleton that is near complete. However, understanding the habitat of these basal hominins has been controversial [4] , [5] . The palaeobiological (partially suggests closed, wooded habitat) [3] , [5] and stable carbon isotopic (indicates wooded grassland habitat) [4] data of the Ar. ramidus bearing the Lower Aramis Member can be reconciled by speculating a riparian (river or lake edge) forest habitat bordered by open, woody grasslands [4] . Fossil assemblage of this riparian strip could indicate closed canopy, which, on the other hand, would be too short lived (because of migrating river channel) and restricted geographically to leave insufficient record in stable carbon isotope of pedogenic (soil forming) carbonate nodules. 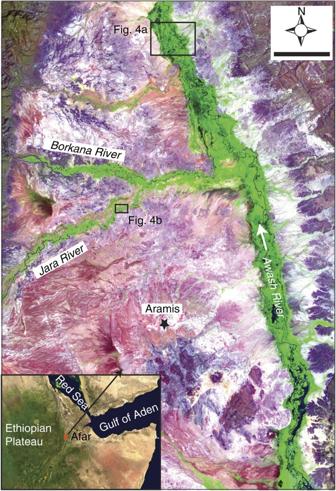Figure 1: Location map. Satellite (ASTER) image showing study area at Aramis surrounded by modern Jara and Awash rivers in Afar, Ethiopia, whereArdipithecus ramidusskeleton (nick name 'Ardi') was discovered1. Afar rift, northernmost part of the East African Rift systems, also famously hosts other important hominin fossils, includingArdipithecus kadabba,Australopithecus afarensis,Australopithecus garhiandHomo sapiens. Note the locations ofFigure 4a,b. Scale bar: 5 km. Figure 1: Location map. Satellite (ASTER) image showing study area at Aramis surrounded by modern Jara and Awash rivers in Afar, Ethiopia, where Ardipithecus ramidus skeleton (nick name 'Ardi') was discovered [1] . Afar rift, northernmost part of the East African Rift systems, also famously hosts other important hominin fossils, including Ardipithecus kadabba , Australopithecus afarensis , Australopithecus garhi and Homo sapiens . Note the locations of Figure 4a,b . Scale bar: 5 km. 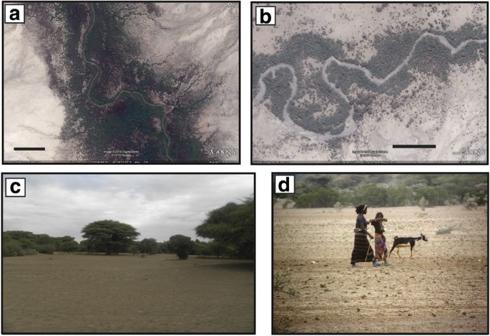Figure 4: Modern floodplains around Aramis, Ethiopia. (a) Modern Awash (scale bar: 500 m) and (b) Jara (scale bar: 200 m) rivers (for locations, seeFig. 1) are associated with narrow corridors of forestland (closed canopy) bordered by more open grassland environments. (c) These riparian corridors (floodplain of Jara) serve as attractive habitats for a number of faunas, including modern Afar tribes (d). We suggest that early hominins inhabited a similar riparian environment at Aramis at 4.4 Myr. Full size image Here we present new sedimentological, palaeohydraulic and palaeosol carbonate-based isotopic evidence for such a riparian environment at Aramis 4.4 million years (Myr) ago. We focus at the site where in-situ Ar. ramidus skeleton (ARA-VP-6/500; nicknamed 'Ardi') was excavated [1] , and present temporally high-resolution (that is, bed scale) sedimentological and isotopic evidence for the environmental context of the very place and time where/when Ardi likely lived and died. Sedimentology Although our sedimentological observation of the Aramis Member of the Sagantole Formation at Ardi excavation site ( Fig. 2 ) broadly matches with the previous work [2] , there are significant differences. We identified previously unrecognized (or not emphasized) two channelized sandstone intervals just below and above the Daam Aatu Basaltic Tuff (DABT), and one un-named, vitric tuff layer ( Fig. 2 ). The channelized sandstone below DABT ( Fig. 2 ) locally erodes into the floodplain deposits containing Ardi skeleton. The upper channelized sandstone erosionally overlies DABT ( Fig. 2 ). Our targeted stratigraphic interval from where sedimentological and stable isotopic data were produced is sandwiched between lower Gaala Tuff Complex and upper Wodara Basaltic Tuff ( Fig. 2 ). Gaala Tuff Complex and DABT have statistically indistinguishable 40 Ar/ 39 Ar dates of 4.4 Myr [2] . Although Wodara Basaltic Tuff is undated, Kullunta Basaltic Tuff (KUBT), yielding a 40 Ar/ 39 Ar age of 4.32 Myr, is located stratigraphically 50 m above the DABT [6] . Although the sediment aggradation rate in a basin can vary in time and space, a linear age interpolation for the deposits between DABT and KUBT, at an average aggradation rate of 0.5 mm yr −1 , suggests that the upper channel-body was likely deposited within 5,000 years after the deposition of DABT, a time span that is within the error margin (±31,000 years) of DABT age [2] . Hence, the palaeorivers that deposited those channelized sandstones likely co-existed with Ar. 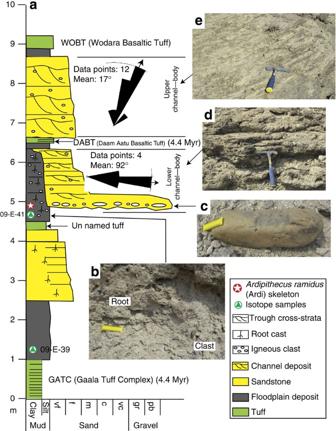ramidus at Aramis, and our study interval has a time span of few thousand to most tens of thousands of years. Figure 2: Sedimentology of the study area. (a) Detailed sedimentological log at Aramis, Ethiopia, the excavation site of the Ardi skeleton, showing two channelized sandstones and their palaeocurrent rose diagrams. Note the40Ar/39Ar ages of marker tuffs2. (b) Floodplain deposits with root casts and scattered igneous clasts. Scale is 5 cm long. (c) A large, well-rounded pebble found at the base of the lower channel body. Dune scale trough cross-strata characterize both lower channel body (d) and upper channel body (e). Figure 2: Sedimentology of the study area. ( a ) Detailed sedimentological log at Aramis, Ethiopia, the excavation site of the Ardi skeleton, showing two channelized sandstones and their palaeocurrent rose diagrams. Note the 40 Ar/ 39 Ar ages of marker tuffs [2] . ( b ) Floodplain deposits with root casts and scattered igneous clasts. Scale is 5 cm long. ( c ) A large, well-rounded pebble found at the base of the lower channel body. Dune scale trough cross-strata characterize both lower channel body ( d ) and upper channel body ( e ). Full size image Both lower and upper channel-bodies consist of predominantly fine-grained sandstones, showing mainly cross-bedding with scattered igneous clasts ( Fig. 2 ). These cross-beddings, with >5 cm thick set, show upper angular contacts and lower tangential contacts. Hence, these are interpreted as dune scale trough cross-stratification. Cross-beddings in the lower channel body have lengths of 50–100 cm and a mean set thickness of 17 cm, whereas those in the upper channel body are >100 cm long with a mean set thickness of 34 cm. Erosional basal lags of the lower channel body contain well-rounded igneous clasts up to 15 cm long, indicating a long-distance sediment transport. The upper channel body also shows scattered igneous clasts, which are up to 3 cm long and well rounded. Notably, numerous granule-size (2–4 mm) igneous clasts are scattered throughout the Ardi skeleton-bearing floodplain deposits, which show relict beddings disrupted by bioturbation ( Fig. 2b ). Similar clasts are also found in the adjacent lower channel body, suggesting that the floodplain was repeatedly flooded by the nearby palaeoriver. Sandstone interval immediately below the un-named tuff is poorly sorted with root casts and no bedwave-type sedimentary structures ( Fig. 2a ), possibly indicating repeated overbank splay deposits resulted from high-energy flows originating from a nearby river. Palaeocurrent analysis of trough cross-strata reveals an eastward (mean 92°) flow for the lower channel body and northward (mean 17°) flow for the upper channel body ( Fig. 2a ). Majority of the floodplain deposits of the studied succession has a massive (that is, unstratified) appearance with distinct pedogenic features like clay cutans, blocky ped structures, root/burrow traces and mottling. These palaeosol horizons contain dispersed to clustered calcareous nodules, which were sampled for stable carbon and oxygen isotope analysis. Palaeohydraulic reconstruction, mainly based on sediment grain sizes and sedimentary structures (see Method and Supplementary Information for details), of the lower and upper channel-bodies suggests that the streams that deposited these channelized sandstones were not small. With a bankfull depth of 4 m and a bankfull width of 110 m, the lower channel was capable of generating a bankfull discharge of 330 m 3 s −1 , whereas with a bankfull depth of 8 m and a bankfull width of 390 m, the upper channel was capable of generating a bankfull discharge of 2540 m 3 s −1 . Although not precise, palaeohydraulic calculations presented here provide a critical first-order approximation of the dimensions and palaeodischarges of the rivers that co-existed (likely within few thousand years) with Ardi at Aramis. However, it is also likely that the lower channel body may represent a crevasse channel of a main river. In any case, our sedimentological data strongly argue for the presence of sizable rivers at 4.4 Myr in the study area. Isotopic analysis Stable carbon and oxygen isotopes preserved in ancient pedogenic carbonate nodules are routinely used to decipher distribution and change of vegetation (that is, C 3 trees versus C 4 grasses) as well as climate change in Cenozoic [7] , [8] , [9] . Several studies [2] , [10] , [11] , [12] from Ardipithecus -bearing Pliocene interval of Afar, Ethiopia linked isotopic values of pedogenic carbonates to the fraction of C 3 versus C 4 vegetation existed at that time. To investigate further the environmental context of Ar. ramidus , we analyzed δ 13 C and δ 18 O of carbonate nodules, collected with targeted sampling from two palaeosol beds ( Fig. 2 ) at the Ardi excavation site at Aramis. The overall low δ 13 C values (‰, Peedee belemnite (PDB)), ranging from −6.28 to −2.26 ( n =8), suggest open woodland with substantial coverage (likely 40 to 80%) of C 4 plants ( Fig. 3 ). Mean 3‰ increase in δ 13 C values, indicating increased presence of C 4 plants, in the upper palaeosol bed compared with the lower palaeosol bed warrants further scrutiny. δ 18 O values of pedogenic carbonates are sensitive to climate (for example, temperature, rainfall, evaporation) and/or altitude [7] , [13] , [14] , a change of which cannot be invoked to explain this increase in C 4 plants, as the mean difference of δ 18 O values (‰, PDB) between the lower and upper palaeosol is only 0.35. Local change of δ 13 C values in pedogenic carbonate linked solely to the shifting belts of C 3 versus C 4 plants in riparian environments due to the migrating streams is well documented [11] , [14] , [15] . In one study at Gona (70 km north of Aramis; Fig. 1 ), this riparian effect is well illustrated in δ 13 C values of vegetation and soil organic matter from adjacent to the modern Awash River, flanked by riparian forest that is bordered by grasslands [11] . In fact, at Gona, δ 13 C values (‰, PDB) of palaeosol carbonates of a Pliocene (2.7 Myr) bed adjacent to a palaeochannel deposit that were interpreted to record riparian mixed vegetation (woody plants and grasses), ranges from −7.6 to −2.0 (ref. 11 ), which is similar to the range of our δ 13 C values. 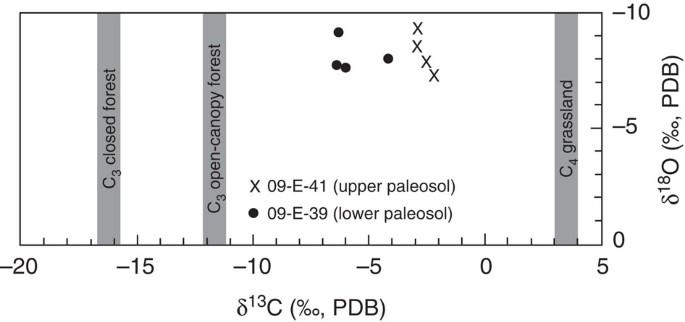Taken together, our δ 13 C and δ 18 O values strongly support for riparian forest to grassland environment at the Ardi excavation site at 4.4 Myr. Figure 3: Carbon and oxygen isotope values of the studied succession. δ13C and δ18O values (‰, PDB) of carbonate nodules, collected with targeted sampling from two palaeosol beds (Fig. 2a) at the Ardi excavation site at Aramis, Ethiopia. Vertical grey bars indicate expected δ13C values of soil carbonates forming under a C4grassland, C3plants in open-canopy forest, and a closed-canopy forest (higher value due to 'canopy effect') during 5.2–3.9 Myr at Gona (70 km north of Aramis;Fig. 1), when corrected for enrichment factor of ancient atmospheric CO2and of plant to soil carbonate12. Our δ13C values reflect overall open woodland setting with substantial presence of C4plants. The high range of δ13C values, in conjunction with the low range of δ18O values, can be indicative of soil carbonate forming beneath a riparian forest to grassland (repeat measurements of the internal laboratory standards yielded precision of 0.03‰ for δ13C and 0.02‰ for δ18O). Figure 3: Carbon and oxygen isotope values of the studied succession. δ 13 C and δ 18 O values (‰, PDB) of carbonate nodules, collected with targeted sampling from two palaeosol beds ( Fig. 2a ) at the Ardi excavation site at Aramis, Ethiopia. Vertical grey bars indicate expected δ 13 C values of soil carbonates forming under a C 4 grassland, C 3 plants in open-canopy forest, and a closed-canopy forest (higher value due to 'canopy effect') during 5.2–3.9 Myr at Gona (70 km north of Aramis; Fig. 1 ), when corrected for enrichment factor of ancient atmospheric CO 2 and of plant to soil carbonate [12] . Our δ 13 C values reflect overall open woodland setting with substantial presence of C 4 plants. The high range of δ 13 C values, in conjunction with the low range of δ 18 O values, can be indicative of soil carbonate forming beneath a riparian forest to grassland (repeat measurements of the internal laboratory standards yielded precision of 0.03‰ for δ 13 C and 0.02‰ for δ 18 O). Full size image Hominin fossil record recovered from floodplain deposits of the Lower Aramis Member at Aramis represents at least 36 individuals of Ar. ramidus , including the in-situ preservation of Ardi skeleton (ARA-VP-6/500) [1] , [3] . At this site, and from a stratigraphic interval spanning few thousand (to at most tens of thousands) years at 4.4 Myr, we identified significant channelized deposits directly adjacent to Ar. ramidus -bearing floodplain strata, which yielded overall low, yet with a large range of, δ 13 C values of pedogenic carbonates, indicating mixed vegetation (woody plants and grasses) in floodplain environment. This suggests that these early hominins inhabited riparian environments, likely taking the advantage of water-fed ecosystems developed in a narrow forest corridor bordered by more open woody grasslands, along the banks of palaeorivers. Modern Jara and Awash rivers near Aramis ( Fig. 1 ) show similar densely vegetated (forestland to woodland) corridors (0.5–1 km wide for Jara and 1–2 km wide for Awash), which are rich in faunas, within a rather dry, grassland landscape ( Fig. 4 ). Figure 4: Modern floodplains around Aramis, Ethiopia. ( a ) Modern Awash (scale bar: 500 m) and ( b ) Jara (scale bar: 200 m) rivers (for locations, see Fig. 1 ) are associated with narrow corridors of forestland (closed canopy) bordered by more open grassland environments. ( c ) These riparian corridors (floodplain of Jara) serve as attractive habitats for a number of faunas, including modern Afar tribes ( d ). We suggest that early hominins inhabited a similar riparian environment at Aramis at 4.4 Myr. Full size image East Africa has been the centre place for human evolutionary studies, including investigation of why and how hominins split off from early apes. Understanding the dynamic nature of the early Pliocene landscape and environments, once frequented by hominins, both at regional and local scale is critical to evaluate the role of physical environment as a driver for hominin evolution [16] . The evidence we presented here for the riparian environmental context of basal hominins at Aramis, Ethiopia 4.4 Myr ago has clear implications for assessing various hypotheses [17] , [18] , [19] related to drivers and mechanisms of early hominin evolution, including the development of bipedalism. Palaeohydraulics Palaeohydraulic calculations are routinely used in interpreting ancient fluvial deposits [20] , [21] , [22] , [23] , [24] , [25] , [26] , [27] , despite some critical challenges [28] , [29] , which are rather generic to quantitative understanding of complex earth surface processes. In particular, recent advancements in palaeohydraulics [24] , [25] , [26] , [27] , [29] allowed us to calculate palaeochannel dimensions and their palaeo discharges from channelized sandstones deposited at 4.4 Myr at Aramis, Ethiopia. We targeted two channelized sandstone intervals just below (henceforth called lower channel) and above (henceforth called upper channel) the DABT ( Fig. 2 ) at the site where Ardipithecus ramidus skeleton (ARA-VP-6/500) was excavated [1] , [2] ( Fig. 1 ). In fluvial deposits, preserved thicknesses of dune-scale cross-sets are specifically useful in estimating channel depth, first by calculating formative dune height and then linking dune height to water depth [23] , [24] , [25] , [26] , [29] , [30] . For this, measurements of dune-scale cross-set thickness (s) were compiled ( Supplementary Table 1 ) to calculate the mean ( s m ) and s.d. ( s sd ). It has been demonstrated that when s sd / s m is closer to 0.88(±0.3), mean dune height ( h m ) can be estimated as [23] , [24] , [25] , [29] : It has also been shown that, for all types of river dunes (including those not in equilibrium with the flow), d / h m averages between 6 and 10, where d is the flow depth [23] , [24] , [25] , [30] . Following these procedures, we calculated flow depths between 3 and 5 m for lower channel, and 6 and 10 m for upper channel ( Supplementary Table S1 ). Assuming that the dunes and cross-strata were formed during bankfull flow conditions, reasonable estimates of the mean bankfull channel depths ( d m ) are 4 m for lower channel and 8 m for upper channel ( Supplementary Table S2 ). Furthermore, for sinuous rivers (that is, sinuosity >1), bankfull channel width ( w ) can be estimated as [31] : Using equation 3, we estimated bankfull channel width of 110 m for lower channel and 390 m for upper channel ( Supplementary Table S2 ). For palaeodischarge estimation, we proceed with this equation: Where Q is discharge, A is channel cross-section area (width× depth) and U is flow velocity. Given that a channel cross-section is not rectangular and rather curved, the actual A is approximately 0.65( w × d m ) ( Supplementary Table S2 ) [27] . Channelized sandstones of the studied successions are predominantly fine-grained sands (0.13–0.25 mm), containing mainly dune-scale cross-strata. These information are useful in estimating U . Specific bedwaves (for example, ripples, dunes) are stable within specific ranges of grain size, flow depth and flow velocity [26] , [32] ( Supplementary Fig. S1 ). For example, existence (not height) of dunes is weekly dependent on flow depth but is strongly dependent on flow velocity and grain size. For lower and upper channels, a range of flow velocities can be estimated from bedwave stability graph ( Supplementary Fig. S1 ) using grain size (fine sand) and previously calculated flow depths. Assuming that sedimentary structures (for example, dune-scale cross-strata) generated during high-stage or immediately after flood-stage are preferentially preserved in the rock record, we determined 1.15 and 1.25 m s −1 as reasonable estimates of high-stage flow velocities for lower and upper channels, respectively ( Supplementary Table S2 ). In this way, we calculated palaeodischarges of 330 and 2540 m 3 s −1 for lower and upper channels, respectively ( Supplementary Table S2 ). Notably, these discharges do not represent mean annual discharge but indicate bankfull discharge, which has a return period of a few years. Although the standard errors of the above estimations are large, and we were able to measure successfully a small population of cross-set thickness (due to limited outcrops), palaeohydraulic calculations presented here provide a critical first-order approximation of the dimensions and palaeo-discharges of the rivers that co-existed with Ardipithecus ramidus at Aramis. Hydraulics of modern Jara and Awash rivers, which flow around Aramis region ( Fig. 1 ), match reasonably well with the lower and upper channels, respectively ( Supplementary Table S2 ). As modern Awash is an incised river [33] , [34] , it has a smaller width/depth ratio compared with the upper channel. Moreover, the upper-channel discharge was expectedly higher because of different tectonic and palaeoclimatic conditions [34] , [35] , [36] . Stable isotopes of pedogenic carbonates Pedogenic calcareous nodules were sampled >50 cm below the upper contacts of palaeosol beds to prevent the influence of 13 C-enriched palaeo-atmospheric CO 2 on δ 13 C values, and to minimize the effect of soil water evaporation on δ 18 O values, of analyzed carbonates. Carbonate nodules were dissected to study under binocular microscope to ensure that diagenetic spars (generally found in veins) were avoided in isotopic analysis. Microsampling of dissected nodules and their isotope analysis were done in the Stable Isotope Laboratory of Tulane University. Using a computer-controlled MicroMill machine, powders of various interior parts of the dissected nodules were sampled. These samples were analyzed by an automated, dual-inlet Isoprime isotope ratio mass spectrometer. Carbon and oxygen isotopic ratios are reported in the standard δ notation as the per mil (‰) difference from the Peedee belemnite international standard (NBS-19). Repeat measurements of the internal laboratory standards yielded precision of 0.03‰ for δ 13 C and 0.02‰ for δ 18 O. Data are presented in Supplementary Table S3 . How to cite this article: Gani, M. R. & Gani, N. D. River-margin habitat of Ardipithecus ramidus at Aramis, Ethiopia 4.4 million years ago. Nat. Commun. 2:602 doi: 10.1038/ ncomms1610 (2011).